A genome-wide map of hyper-edited RNA reveals numerous new sites Adenosine-to-inosine editing is one of the most frequent post-transcriptional modifications, manifested as A-to-G mismatches when comparing RNA sequences with their source DNA. Recently, a number of RNA-seq data sets have been screened for the presence of A-to-G editing, and hundreds of thousands of editing sites identified. Here we show that existing screens missed the majority of sites by ignoring reads with excessive (‘hyper’) editing that do not easily align to the genome. We show that careful alignment and examination of the unmapped reads in RNA-seq studies reveal numerous new sites, usually many more than originally discovered, and in precisely those regions that are most heavily edited. Specifically, we discover 327,096 new editing sites in the heavily studied Illumina Human BodyMap data and more than double the number of detected sites in several published screens. We also identify thousands of new sites in mouse, rat, opossum and fly. Our results establish that hyper-editing events account for the majority of editing sites. RNA editing is a frequent post-transcriptional modification that leads to nucleotide changes at specific locations. As such, it can be detected directly by sequencing, allowing large-scale screening of editing events. Adenosine-to-inosine (A-to-I) editing is the most common form of editing in mammals, and is catalysed by the adenosine deaminases ADAR1 and ADAR2 proteins, whose target is double-stranded (ds) RNA [1] , [2] , [3] , [4] . Alu repeats are short (≈300 bp) mobile elements widespread in primates, with over a million copies in the human genome. Due to their density, nearby Alu repeats of reverse orientation are common, and if transcribed, can form dsRNA. Therefore, adenosines in inverted pairs of Alu repeats are the majority of known RNA-editing sites, where they are edited irregularly [5] , [6] , [7] , [8] , [9] . Consistent editing of a handful of coding nucleotides is also known, with the editing of some sites being essential. Recently, the effect of RNA editing has been gradually elucidated and its connections to various diseases have been established [10] , [11] , [12] . It is, therefore, of importance to be able to accurately detect RNA editing in a sample. Naively, detection of editing sites in RNA-seq data should be straightforward, because sequencing of an edited cDNA will read edited adenosines (A) as guanosines (G). Thus, by simply aligning RNA-seq reads to the reference genome and searching for A-to-G mismatches, one should easily detect editing sites. Several computational schemes have exploited this idea, with increasing levels of success [9] , [13] , [14] , [15] , [16] , [17] , [18] . However, there are several other sources of discrepancies between RNA-seq reads and the reference DNA, making the identification of genuine editing events challenging. Confounders include sequencing errors, polymorphisms and, most importantly, an incorrect alignment of the RNA-seq reads to their genomic location. Specifically, it was found that careful alignment is necessary to reduce systematic errors due to ‘alignment hazards’, such as duplications, splicing, repeats and pseudogenes. To maintain high standards of alignment, current approaches allow only a small number of mismatches between the reads and the genome (these mismatches later become editing site candidates). Thus, although it is well known that ADAR tends to edit sites in clusters (‘hyper-editing’) [5] , [6] , [8] , [19] , [20] , [21] , [22] , current methods miss the heavily edited short reads. Here, we present an approach that overcomes this obstacle (by pre-masking potential A-to-G-editing sites in unaligned reads [19] ) and enables the large-scale detection of hyper-edited reads in RNA-seq studies. By applying our approach to a number of recent (human and non-human) RNA-seq data sets, we show that our method discovers, with high specificity, a much larger number of editing sites than previous RNA-editing detection approaches, in some cases by orders of magnitude. Our results thus establish that screening for hyper-editing is crucial in order to obtain a reliable picture of RNA editing. Detecting hyper-edited reads in RNA-seq data Editing detection methods rely on mapping RNA sequences to the genome using tools that allow only a limited number of mismatches. This prevents the mapping of hyper-edited (short) reads, and therefore, their editing sites go undetected. To identify extensively edited regions, we apply a simple but effective four-step approach: (1) collect all unmapped reads from the initial alignment; (2) transform all As to Gs in both the unmapped reads and the reference genome; (3) realign the transformed RNA reads and the transformed reference genome; and (4) recover the original sequences and search for dense clusters of A-to-G mismatches. An overview of the pipeline is presented in Fig. 1 ; complete details are provided in Methods. 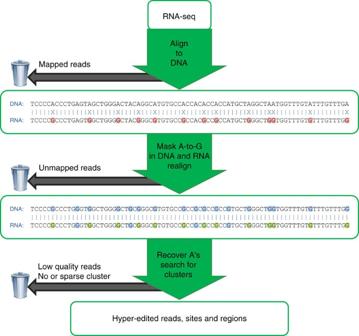Figure 1: Overview of our hyper-editing detection pipeline. In the first step, an RNA-seq data set is aligned to the reference genome and mapped reads are discarded. Hyper-edited reads do not map in this step since they contain too many mismatches (see a hypothetical example in the top alignment; edited nucleotides highlighted in red). To detect potential RNA editing in the unmapped reads, we realign them after masking the editing sites by transforming all As to Gs in both RNA and DNA (bottom alignment; transformed nucleotides in blue, edited nucleotides in green). For those reads that realign, the original sequences are recovered and examined for high-quality clusters of A-to-G mismatches. Reads with large, dense clusters of A-to-G differences are designated as hyper-edited, and their editing sites are recorded. See complete details in Methods. Figure 1: Overview of our hyper-editing detection pipeline. In the first step, an RNA-seq data set is aligned to the reference genome and mapped reads are discarded. Hyper-edited reads do not map in this step since they contain too many mismatches (see a hypothetical example in the top alignment; edited nucleotides highlighted in red). To detect potential RNA editing in the unmapped reads, we realign them after masking the editing sites by transforming all As to Gs in both RNA and DNA (bottom alignment; transformed nucleotides in blue, edited nucleotides in green). For those reads that realign, the original sequences are recovered and examined for high-quality clusters of A-to-G mismatches. Reads with large, dense clusters of A-to-G differences are designated as hyper-edited, and their editing sites are recorded. See complete details in Methods. Full size image We previously introduced and applied an early version of this approach to detect hyper-edited human ESTs (expressed sequence tags) [19] . Other groups have recently employed similar approaches to study editing in Drosophila melanogaster [23] and Caenorhabditis elegans [24] . Here, we describe the results of an extended and improved pipeline that is aimed at detecting hyper-editing in RNA-seq data. In contrast to our previous method, the new pipeline addresses the challenges associated with the numerous and much shorter sequences derived from RNA-seq data, such as ambiguously aligned reads, incorrect mapping due to splicing, paired-end (PE) reads and homopolymeric sequences (see Methods for more details). The main data set we considered was the Illumina Human BodyMap 2.0, consisting of ≈5 × 10 9 reads (of lengths 50, 75 and 100 bp), of which ≈788 × 10 6 reads remained unmapped after running BWA. After some initial filtering (Methods), we applied our pipeline to detect hyper-edited reads, defined here as reads with ≥5% density of high-quality A-to-G mismatches (Method s ). Note that we did not attempt to discover moderately edited reads, as those are usually mapped in the first step and thus not considered by our pipeline. Our final hyper-editing set consisted of 637,426 reads, containing 649,756 unique A-to-G-editing sites. In the remainder of the paper, we report the analysis of hyper-editing in the 75-bp subset of the Illumina BodyMap data consisting of ≈1.3 × 10 9 single-end (SE) reads, of which ≈114 × 10 6 reads were unmapped. We discovered 390,881 hyper-edited reads ( Supplementary Data 2 ), containing 455,014 unique A-to-G-editing sites ( Supplementary Data 1 ) (2,080,519 in total) at 62,860 distinct regions ( Fig. 2a and Supplementary Table 1 ; see Methods for definitions). For comparison, careful screening for editing in the pool of the mapped reads in the Illumina BodyMap data was previously carried out by Ramaswami et al . [17] These authors detected (in the 50 and 75 bp data sets) 370,623 sites, but only 59,361/455,014 (13.0%) of the sites that we detected when we used a subset of the same data (namely, the 75-bp data set). These results suggest that extensive editing by ADAR enzymes is not only highly abundant but also missed by existing computational screens. 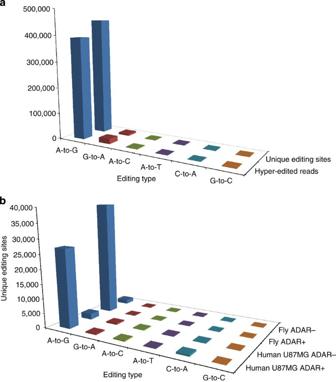Figure 2: Counts of hyper-editing events. (a) Hyper-editing identified in the Illumina BodyMap 75-bp SE read set. Most of the detected hyper-edited reads (390,881/414,898; 94.2%) were of A-to-G type. A total of 455,014 unique A-to-G-editing sites were discovered, 97.2% of all the detected unique sites. (b) Most editing sites were eliminated in ADAR− samples. We detected hyper-editing sites inDrosophilanascent-RNA-Seq data from either wild-type (ADAR+) flies or from ADAR-null (ADAR−) flies. The number of A-to-G sites detected in the ADAR+ sample was ≈20-fold larger than in the ADAR− sample (39,472 versus 1,436; there were 2 × 10−4editing sites per (mapped) read in ADAR+ compared with 9 × 10−6in ADAR−). Similarly, we detected hyper-editing sites in the human U87MG cell line, either with (ADAR−) or without (ADAR+) siRNA-induced silencing of ADAR1. The number of sites in the ADAR+ sample was much higher than in the ADAR− sample (27,124 versus 1,992, or 3 × 10−4versus 2 × 10−5sites per mapped read). The number of non-A-to-G-editing sites is also presented. In the ADAR+ samples, more than 94% of the detected sites were A-to-G. In the ADAR− samples, while the number of A-to-G sites significantly decreased, the counts of the other mismatches were almost indifferent to the absence of ADARs. Figure 2: Counts of hyper-editing events. ( a ) Hyper-editing identified in the Illumina BodyMap 75-bp SE read set. Most of the detected hyper-edited reads (390,881/414,898; 94.2%) were of A-to-G type. A total of 455,014 unique A-to-G-editing sites were discovered, 97.2% of all the detected unique sites. ( b ) Most editing sites were eliminated in ADAR− samples. We detected hyper-editing sites in Drosophila nascent-RNA-Seq data from either wild-type (ADAR+) flies or from ADAR-null (ADAR−) flies. The number of A-to-G sites detected in the ADAR+ sample was ≈20-fold larger than in the ADAR− sample (39,472 versus 1,436; there were 2 × 10 −4 editing sites per (mapped) read in ADAR+ compared with 9 × 10 −6 in ADAR−). Similarly, we detected hyper-editing sites in the human U87MG cell line, either with (ADAR−) or without (ADAR+) siRNA-induced silencing of ADAR1. The number of sites in the ADAR+ sample was much higher than in the ADAR− sample (27,124 versus 1,992, or 3 × 10 −4 versus 2 × 10 −5 sites per mapped read). The number of non-A-to-G-editing sites is also presented. In the ADAR+ samples, more than 94% of the detected sites were A-to-G. In the ADAR− samples, while the number of A-to-G sites significantly decreased, the counts of the other mismatches were almost indifferent to the absence of ADARs. Full size image The hyper-editing detection screen is highly specific The specificity of an editing detection screen is usually gauged by rerunning the same pipeline, but when looking for dense clusters of mismatches other than A-to-G [5] , [6] , [8] , [20] . Since non-A-to-G editing is expected to be extremely rare [25] , [26] , [27] , the fraction of A-to-G clusters to all clusters represents a useful measure of the screen’s specificity (note that for data sets where the sequenced strand is random, such as the 75-bp subset of the BodyMap, when we refer to A-to-G-editing sites, they may actually be either A-to-G or T-to-C). Our screen for hyper-editing in the Illumina BodyMap data achieved high specificity, with 97.25% of the unique hyper-editing sites being A-to-G ( Supplementary Table 1 ), higher than in previous screens of other data sets (summarized in Table 1 in ref. 16 ; when not limited to Alu ). Beyond A-to-G, the other mismatch type with the most hyper-editing sites was G-to-A, with only 1.64% of the total number of unique editing sites (7,664/467,894) ( Fig. 2a and Supplementary Table 1 ). Even this remarkable low level of noise is likely an overestimate, since a few of the G-to-A events may be genuine DNA or RNA editing by APOBEC proteins [28] , [29] , [30] . The ratio of A-to-G to G-to-A hyper-edited reads was 20.4, compared with 59.4 for the ratio of A-to-G to G-to-A unique-editing sites ( Supplementary Table 1 ), suggesting that many G-to-A events are concentrated at a small number of likely erroneous sites. Additionally, A-to-G sites overlapping with a known genomic SNP (single-nucleotide polymorphism), which are unlikely to be true editing sites [31] , were just 1.64% of all sites, much less than for the other mismatch types ( Supplementary Table 1 ). Finally, even more support for the specificity of our method comes from the strand information. The RNA-seq data we used (the 75-bp reads subset) is strand-indifferent, and therefore, even for true A-to-G sites, the observed mismatches are either A-to-G or T-to-C with roughly equal amounts ( Supplementary Fig. 1 ). However, the Illumina BodyMap project also contains a data set of strand-informative 100-bp reads, in which the sequenced strand is identical to the expressed strand. In that data set, A-to-G is the only type of mismatch that is (almost) exclusively found on the expressed strand ( Supplementary Fig. 1 ), suggesting that other ‘editing’ types are due to technical errors. Similarly, in 191,774/225,879 (84.9%) of the A-to-G 75-bp hyper-edited reads that intersected with RefSeq sequences, the sense strand mismatch was A-to-G (compared with 3,832/9,495 (40.4%) for G-to-A hyper-edited reads). The remaining A-to-G edited reads (15.1%) may be due to editing of transcripts expressed from the antisense strand [32] , [33] . Table 1 Published methods discard the vast majority of editing sites. Full size table Most of the detected editing sites are novel The majority of the editing sites detected by our method were novel. Of 455,014 unique sites, only 42,775 (9.4%) and 126,983 (27.9%) appeared in DARNED [34] (total 322,415 sites) and RADAR [35] (total 1,379,403 sites), respectively, the latter supposedly being the most comprehensive database of human RNA editing to date. The number of sites that are novel with respect to both databases is 327,096/455,014 (71.9%) and the number of novel regions (not containing any known editing sites) is 25,170/62,860 (40.0%). Our results, therefore, suggest that the majority of our detected regions—precisely those that are most excessively edited—are missed by traditional approaches. Sequence context and tissue of origin of hyper-editing sites Examining the sequence context of our detected sites showed that Gs are depleted one base upstream and enriched one base downstream of the editing sites ( Fig. 3 ), in agreement with the known ADAR sequence preference [36] and the known ADAR targets [17] , [37] . In order to study differential hyper-editing among tissues, we assigned each tissue an enrichment factor based on its relative editing level (see details in Supplementary Table 2 ). The brain had the highest enrichment factor, as well as the largest number of unique hyper-edited regions and sites, consistently with previous studies [5] , [6] , [20] , [38] . Interestingly, the brain did not have a particularly large number of hyper-edited reads ( Supplementary Table 2 ), suggesting that while editing in the brain encompasses more hyper-editing sites than in other tissues, many of them are expressed and/or edited to low levels. 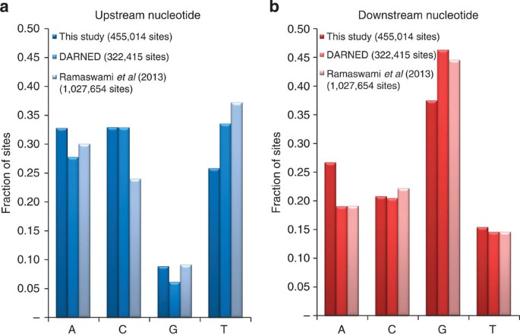Figure 3: Sequence context of hyper-editing. The bars correspond to the fraction of editing sites with each type of (genomic) nucleotide one base (a) upstream and (b) downstream of the site. Results are shown for sites from our study, the DARNED database, and Ramaswamiet al.17The sequence near the hyper-editing sites is depleted of Gs upstream and enriched with Gs downstream. Figure 3: Sequence context of hyper-editing. The bars correspond to the fraction of editing sites with each type of (genomic) nucleotide one base ( a ) upstream and ( b ) downstream of the site. Results are shown for sites from our study, the DARNED database, and Ramaswami et al . [17] The sequence near the hyper-editing sites is depleted of Gs upstream and enriched with Gs downstream. Full size image Genomic localization of hyper-edited regions The majority of the hyper-edited regions overlapped with genes (41,531/62,860; 66%), usually with introns (38,534/41,531; 93%). As previously found for most editing targets [5] , [6] , [8] , [20] , hyper-edited regions localized mostly in Alu repeat elements (55,106/62,860; 88%). These Alu repeats likely form a dsRNA structure, the ADAR target, by hybridizing with nearby, oppositely oriented Alu s. Only 3,539/62,860 regions (5.6%) did not overlap with any documented repetitive element (see more below). Coding and microRNA-related hyper-editing sites To detect coding hyper-editing sites, we used the RefSeq annotation as well as additional filtering of genomic SNPs and A-to-G mismatches that were not on the (RefSeq-annotated) expressed strand. Overall, we detected 728 coding sites ( Supplementary Data 3 ) in 140 genes (out of a total of 32,693 exonic sites), of which 507 were non-synonymous and three were non-stop (Annovar [39] ). These coding hyper-editing sites exhibited the known ADAR motif (depletion of G one base upstream of the site), but with a somewhat weaker magnitude (not shown). Only 75 of the coding sites (48 of the non-synonymous) appeared in RADAR [35] . Editing of microRNAs (miRNAs) or their precursors may impact miRNA maturation and function [40] . Our analysis of the BodyMap data predicted 20 novel editing sites (total 29; Supplementary Data 4 ) in six primary transcripts of known miRNA (miRBase [41] ), with 11 novel sites (total 14) localized in five mature miRNA regions. Moreover, we detected 61 new editing sites in conserved mammalian miRNA regulatory targets in 3'–untranslated regions (predicted by TargetScanHuman [42] ). Pinto et al . [43] reported 59 evolutionary conserved mammalian-editing sites in 33 genes. While we detected only two of these sites, we detected additional 505 hyper-editing sites in 20 out of these 33 genes (only 150 of which were in RADAR), 1.6-fold more than in all other genes (8,678/23,000). This supports the hypothesis that hyper-editing can induce site-selective editing [44] . Hyper-edited Alu s are part of long dsRNA structures Our previous, smaller-scale study of hyper-editing in ESTs found that hyper-edited Alu s are predicted to form particularly stable dsRNA, more than in selectively edited RNAs. To explore whether a similar trend exists here, we compared the 49,264 hyper-edited Alu s to 234,503 Alu s that were identified as edited [17] but were not hyper-edited. Indeed, the average distance between a hyper-edited Alu and the nearest inverted Alu (814±1,103 bp) was significantly shorter than in moderately edited Alu s (1,130±1,449 bp; P <10 −300 ; Wilcoxon rank-sum test). The maximal number of pairs of inverted Alu repeats flanking an edited Alu (±10 kb; see Supplementary Fig. 2 for definition) was significantly higher in hyper-edited Alu s (8.13±4.60) compared with moderately edited Alu s (7.28±4.54; P <10 −300 ; Wilcoxon rank-sum test). Taken together, these results confirm that hyper-edited Alu s are predicted to be part of longer and more stable dsRNA than moderately edited Alu s ( Supplementary Fig. 2 ). Accuracy of hyper-edited regions outside known repeats The 3,539 hyper-edited regions (containing 29,428 unique sites) that were outside of any known repeat (using RepeatMasker; see Methods) were particularly intriguing, and we attempted to determine whether they were truly hyper-edited or false positives of our method. We assessed the accuracy of editing detection in these regions by three measures: comparison of the number of A-to-G editing events with other types of ‘editing’, the sequence context, and the ability to form a dsRNA structure. A-to-G-editing sites were 77.4% of the total number of sites discovered outside known repeats (29,428/38,033). While this fraction is low compared with the genome-wide value (≈97%), it is one of the highest rates achieved at regions outside known repeats (summarized in Table 1 in ref. 16 ). Next, the A-to-G sites in these regions exhibited the known ADAR motif (depletion of Gs one base upstream; not shown). Finally, we tested for potential formation of long dsRNA structure, the main target of ADARs, by aligning (using bl2seq [45] ) the hyper-edited regions and their flanking (±10 kb) antisense sequences (see Methods). In 33.2% of the hyper-edited regions (1,174/3,539), a match was found (defined as an identity along ≥80% of the region), compared with only 4.5% (161/3,539) of the regions when aligning to the same flanking sequences but on the same strand (in which case dsRNA cannot form). An example of a dsRNA structure predicted in a region outside known repeats is shown in Fig. 4 . Validation, by Sanger sequencing, of editing in this region in an independent brain sample is described in Methods and Supplementary Fig. 3a . In summary, despite the higher noise level at regions outside known repeats, strong evidence suggests that at least the majority of these regions are truly edited. In fact, some of our detected hyper-edited regions may be true repetitive elements missed by current repeat annotation methods. 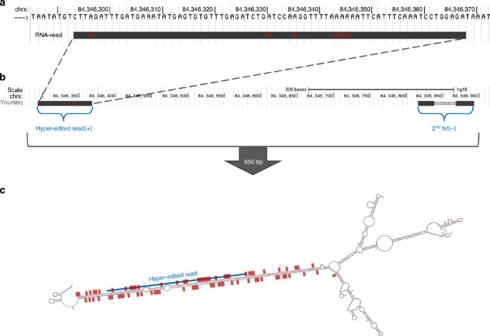Figure 4: Hyper-editing in a region outside known repeats. (a) An alignment of a hyper-edited read to a DNA region outside known repeats. (b) A BLAT search66(The UCSC Genome Browser62), using the hyper-edited read as a query, returned two hits in an opposite orientation: one at the hyper-edited region and another ≈650 bp away, allowing the potential formation of dsRNA. (c) Prediction of the secondary structure of the entire 650-bp region (mfold67). The blue line shows the location of the hyper-edited read ofa; red dots are located at editing sites detected along the entire 650-bp region (both from the read shown ataas well as from other reads). All editing sites are lined along a dsRNA structure. Experimental validation of many of those predicted editing sites is described in Methods and inSupplementary Fig. 3a. Figure 4: Hyper-editing in a region outside known repeats. ( a ) An alignment of a hyper-edited read to a DNA region outside known repeats. ( b ) A BLAT search [66] (The UCSC Genome Browser [62] ), using the hyper-edited read as a query, returned two hits in an opposite orientation: one at the hyper-edited region and another ≈650 bp away, allowing the potential formation of dsRNA. ( c ) Prediction of the secondary structure of the entire 650-bp region (mfold [67] ). The blue line shows the location of the hyper-edited read of a ; red dots are located at editing sites detected along the entire 650-bp region (both from the read shown at a as well as from other reads). All editing sites are lined along a dsRNA structure. Experimental validation of many of those predicted editing sites is described in Methods and in Supplementary Fig. 3a . Full size image 40% of hyper-edited regions are not expressed as unedited We determined, for each of the 103,839 (non-unique; Supplementary Table 2 ) hyper-edited regions detected in all tissues, whether they were covered by reads in the original, strict mapping. We found, somewhat surprisingly, that as many as 40.3% of the hyper-edited regions (41,873) were not covered by even a single read. In other words, these regions were not expressed as unedited or even lightly edited. We speculate that this is the result of these regions being edited so excessively, that the chances of sampling an unedited (or little edited) molecule are extremely small. Alternatively, these regions may be particularly hard to sequence and map. Whatever the reason is, this result highlights the fact that a large fraction of the hyper-edited reads would be completely missed by traditional approaches, as we discuss next in more detail. Published methods discard the vast majority of editing sites Computational editing detection screens usually begin by aligning the RNA sequences to the reference genome. However, as explained above, most published methods, in order to eliminate noisy reads, allow only a handful of mismatches (for example, three mismatches in ref. 15 ; three or four mismatches in ref. 18 ) and thus do not allow the detection of more heavily edited molecules. We showed above, as a proof-of-concept, that hyper-editing can be detected and is highly abundant in the Illumina BodyMap data. Here, we apply our detection pipeline in comparison with nine published RNA-seq data sets (from six publications; including the BodyMap data), where editing sites were previously identified by other groups. The results ( Table 1 ) are remarkable: in all cases, our screen dramatically increased the number of detected sites. Compared with the most comprehensive other studies [17] , we more than doubled the number of editing sites. Compared with the ENCODE study [15] , we strikingly detected 148 times more editing sites. The specificity of our screen (the number of A-to-G-editing sites divided by the number of sites of all types of mismatches) was high, at 94.6% or higher, and the overlap between the sets of previously detected sites and the hyper-edited sites was usually small (at most 62%). As expected [19] , the number of detected hyper-editing sites generally increased with the total number of reads. Taken together, these results suggest that screening for hyper-editing is absolutely crucial for editing detection, or otherwise the majority of sites are overlooked. These two approaches are complementary, that is, both the traditional approach (searching for moderately edited reads) and our approach (screening unmapped reads for hyper-editing) are required to fully characterize the editing spectrum. Alternatively, a new pipeline that combines these two approaches should be developed, based on more sensitive aligners. Identification of hyper-edited RNAs in other species We next applied our editing detection screen to published RNA-seq data sets from mouse, rat, opossum, fly and platypus [46] , [47] , [48] , [49] and detected, with high specificity, thousands of editing sites (11,849, 21,761, 1,563 and 39,472, respectively; nearly no editing sites were detected in the platypus brain) ( Table 2 ) [48] . As in the human data sets, most of the sites we discovered were previously unknown, highlighting the importance of screening for hyper-editing. The mouse and fly data sets have been previously screened for editing, but not for hyper-editing [17] , [23] , [46] , [49] , and we have dramatically increased the number of editing sites in these species. In rat and opossum, we are the first to screen an RNA-seq data set and report thousands of editing sites. To compare the frequency of editing across species, we computed, for each data set, the number of editing sites per mapped read as an approximation of the true editing rate ( Table 2 ). The human editing level was ≈10-fold higher than in non-humans [50] ; the other three mammals we examined had a similar editing rate, while the rate in fly was ≈50% higher. Table 2 Identification of hyper-edited RNAs in different species. Full size table Lack of hyper-editing in ADAR1 knockdown RNA-seq Finally, we applied our hyper-editing detection pipeline to RNA-seq from human and fly cells in which the editing enzymes (ADAR1 and ADAR, respectively) were eliminated ( Fig. 2b ). Such an experiment can serve two purposes: (i) validate that the hyper-editing sites discovered by our method are indeed due to editing by ADAR; and (ii) (in humans) determine the contribution of specific ADAR proteins to hyper-editing. We first analysed nascent RNA from fly heads [49] , from either wild-type or ADAR-null mutant flies (there is a single ADAR protein in Drosophila ). The near-complete elimination of hyper-editing from the ADAR-null sample supports the identification of our discovered sites as true products of editing by ADAR ( Fig. 2b ). We then considered human RNA-seq data from the U87MG cell line, with or without siRNA-induced silencing of ADAR1 (ref. 14 ). The reduction in ADAR1 fragments per kilobase per million mapped reads (FPKM) decreased from 44.01 and 42.72 in the two control samples to 6.17 and 5.33 in the siRNA samples; ADAR2 FPKM decreased from 3.71 and 3.88 to 1.98 and 2.04) eliminated most of the hyper-editing sites, suggesting that hyper-editing is catalysed mostly by ADAR1. Editing events that result in isolated codon changes have been the focus of intensive research in the past two decades. However, recent studies pointed out that most ADAR activity takes place in clusters [6] , [9] , [22] , [51] . In this paper, we implemented an algorithm (improving on our previously published approach [19] ) to detect hyper-edited reads from large-scale RNA-seq data. We showed that our method is highly specific and that the detected sites have the known features of ADAR targets, such as a sequence motif, dsRNA structure, and localization mostly in Alu elements. In humans, we discovered about half a million new sites, a few hundreds of them recoding and hence of particular interest. In other species, we discovered thousands of sites, in some species for the first time on such a large scale. The enormous number of editing sites that we discovered were missed by the traditional approaches, even though, by definition, those sites are located in the most heavily edited regions of the genome. These results suggest that our procedure should be made an integral component of any editing screen. While it is easy to understand the functional consequences of an amino-acid change on the protein product of a gene, the biological impact of hyper-edited regions is less intuitive, specifically as most hyper-editing sites reside in introns and are therefore limited to pre-mRNA. Several studies implicated hyper-edited transcripts in cellular functions that involve, for example, their nuclear retention or degradation [52] , [53] , [54] , [55] , [56] , [57] . One of the most studied mechanisms showed that hyper-edited RNAs bind a protein complex that is largely consist of components of cytoplasmic stress granules, including ADAR1 and Tudor-SN (tudor staphylococcal nuclease) [56] , [58] , [59] . Hyper-edited RNAs then interact with Tudor-SN, which promotes their cleavage [55] . Surprisingly, hyper-edited dsRNAs have also been shown to downregulate both endogenous and reporter gene expression in trans by having global activity to reduce gene expression and inhibit translation initiation [56] . Hyper-edited RNAs are also sufficient to suppress interferon induction and apoptosis in mammalian cells [60] , suggesting that they play an important role in stress response. Finally, a large number of editing events may alter the local dsRNA structure, which, in turn, will have an impact on the ability of the edited RNA to bind other RNAs or RNA-binding proteins. A pre-requisite to a more thorough investigation of any of these mechanisms is the precise identification of the hyper-edited regions. The data set of hyper-edited regions we created addresses this need. For species, tissues, or conditions we did not cover, our method can be applied using our publicly available code. We note that our method is complementary to traditional approaches and is designed to identify only sites in hyper-edited regions. Additionally, our final detected set is sensitive to the precise alignment procedure used. Other parameters that influence the final results are the minimum number of A-to-G differences and the quality score required to call hyper-edited reads, as well as the parameters of the various filters used to remove false positives. There are, therefore, many editing sites that likely escaped our detection. Also, we note that our approach does not provide an estimate of the editing level at each site, which is probably rather low in most cases, and for that purpose, one may use the detected sites as an input to other tools, such as REDITools [61] . Even with those limitations, we discovered a considerable number of sites. However, with ever increasing sequencing depths, the picture emerging from recent studies is that virtually every adenosine in a dsRNA-forming Alu can be edited (although usually at very low levels) [9] . Hence, future studies of RNA editing are expected to shift from mere discovery of editing sites to understanding of editing regulation and function. To this end, hyper-edited RNAs will be important as the result of the most extreme editing process. Therefore, the importance of our method for future research goes beyond the discovery of additional sites, and lies in making possible the characterization of this important class of edited sequences. The pipeline scripts are available at http://levanonlab.ls.biu.ac.il/resources/zip . Data sets The Illumina Human BodyMap 2.0 data set (Gene Expression Omnibus accession code GSE30611 ) consists of ≈5 × 10 9 reads generated from 16 tissues. Each tissue was sequenced at both 50-bp PE reads and 75-bp SE reads. These sets were polyA selected, generated with random priming and not stranded. RNA from a mixture of the same 16 tissues was also sequenced, at 100 bp SE reads, and stranded. The majority of our analysis was carried out on the 75-bp reads data set (≈1.3 × 10 9 ). Identifying hyper-edited reads To find hyper-edited reads, we first aligned all reads (≈5 × 10 9 ) to the human reference genome (hg19) using BWA aln 0.6.2 (default parameters) and mem 0.7.4 (minimum seed length 50). We then considered the unmapped reads, ≈788 × 10 6 in the entire data set and ≈114 × 10 6 in the 75-bp SE data set. While most of the unmapped reads probably represented sequencing artifacts and polymorphisms, we hypothesized that many reads were unmapped due to excessive A-to-G editing [19] . We removed reads with potential sequencing errors [19] : particularly large (>60%) or small (<10%) percentage of a single nucleotide, more than 10% of ambivalent nucleotides (non-(ACGT)), long stretches of simple repeats (>10 repeats, or >20 for a single nucleotide) or an average Phred quality score below 25 (after removing the lowest 10% of the scores). In order to be able to realign reads with a large number of mismatches caused by A-to-G-editing sites, we transformed every A to G in both the remaining RNA reads and in the genome. We aligned the transformed reads to the transformed genome, again using BWA aln 0.6.2 (maximum edit distance 2, no gaps allowed and iterative mode). The original (four-letter) sequences of the reads that aligned (after the transformation) were recovered and the mismatches between the reads and the reference genome were examined. Note that using the original full sequences again eliminates the problem of lower sequence complexity (and hence, lower alignment accuracy) in the transformed reads. Reads that mapped to multiple locations were separately treated by selecting the location with the largest fraction of A-to-G to all mismatches, provided that this fraction was ≥10% higher than in all other locations (otherwise the read was discarded; the read was also discarded if it mapped to >50 locations). We then searched for dense clusters of high-quality (Phred ≥30) A-to-G mismatches, in which the number of A-to-G mismatches was ≥5% of the read length and >60% (80% for read lengths ≤60 bp) of the total number of mismatches. As an additional filtering step, we considered the portion of the read bound by the first and the last A-to-G mismatches. We discarded potentially low-quality/mismapped reads having (i) a too dense A-to-G mismatch cluster (length <10% of the read length); (ii) a cluster too close to the ends of the read (completely contained within either the first or last 20% of the read; those clusters may result from improper alignment to the genome due to splicing); or (iii) a cluster with a particularly large percentage (>60%) of a single nucleotide. For edited PE reads (which were treated throughout the pipeline as two separate single-end reads), we also required that the mate read was mapped to a nearby region (500 kbp) and in an opposite orientation. Reads that passed all filters were finally designated as hyper-edited. An overview of the pipeline is presented in Fig. 1 . In order to determine the pipeline’s specificity, we repeated it when searching for other types of editing events (for example, A-to-C, G-to-A and so on) [19] , which involved modifying the transformation and the definition of the editing mismatches accordingly, but was otherwise identical to the A-to-G screen. There are 12 possible single-nucleotide mismatches. However, since the RNA-seq reads could be either sense or antisense, we could not distinguish between a given mismatch and its complementary one. For example, our detected A-to-G edited reads represent both clusters of A-to-G mismatches and clusters of T-to-C mismatches. The same is true for the other mismatch types, and we therefore report results for only six categories of editing events. For the subset of the Illumina BodyMap containing the 100-bp reads, we again ran the same pipeline. However, since the 100-bp data set was stranded, we could treat A-to-G and T-to-C mismatches separately ( Supplementary Fig. 1 ). Comparison with a previous approach The method proposed here is a natural follow-up of an approach we previously developed to detect hyper-editing in EST libraries [19] , in that it detects editing by realigning hard-to-map reads through masking of potential editing sites. However, the present method was reimplemented from the ground up to address the specific difficulties associated with next-generation sequencing data, where reads are numerous and much shorter. Our remodelled pipeline includes a new and much faster aligner (BWA, reducing running time of the whole pipeline by over 1,000-fold), fine tuning of the parameters of existing filters and introduction of several new pre- and post-processing steps designed for short read data. The new pipeline improves the processing of reads that were aligned to more than one region, takes advantage of information in PE reads and per-base-pair sequencing quality, and filters out reads with potential incorrect mapping at splice sites or with decreasing quality at the ends. We successfully applied our new method to a large number of RNA-seq data sets from several species, and detected several orders of magnitude more sites than was possible with the previous approach. The implementation of our new pipeline has been made public, and is expected to be used for analysing the constantly growing number of RNA-seq data sets. Annotations We annotated genomic regions using RefSeq for known genes and RepeatMasker for known repeats, both from the UCSC Genome Browser [62] downloaded in April 2013. To detect sites overlapping with SNPs, we used genomic SNPs from dbSNP135 (The UCSC Genome Browser). Non-coding RNAs ( Supplementary Data 1 ) were annotated using GENCODE v16. Functional annotation of the predicted editing sites in coding regions was done using ANNOVAR [39] . Human miRNA coordinates were taken from miRBase v20, downloaded from http://www.mirbase.org/ftp.shtml [41] . The coordinates of the conserved mammalian miRNA regulatory targets of conserved miRNA families in the 3'-untranslated regions were predicted by TargetScanHuman v.5.1 (ref. 42 ) (also obtained from the UCSC Genome Browser). Defining hyper-edited regions and dsRNA structure As explained above, we define the cluster of editing mismatches as the portion of the edited read from the first to the last (high quality (Phred ≥30)) A-to-G mismatch. To identify the hyper-edited regions, we first merged (the corresponding genomic coordinates of) all overlapping edited clusters, and then set the boundaries of the region from the first base of the most upstream cluster to the last base of the most downstream cluster. Construction and analysis of the edited regions were carried out using BEDTools [63] . To detect potential dsRNA structure formed by hyper-edited RNAs, the DNA sequences of the hyper-edited regions were aligned to the sequences 10 kbp upstream and 10 kbp downstream of the regions. We used bl2seq [45] with parameters -F F -W 7-r 2, and considered a match only for alignment with 90% identity along 80% of the hyper-edited region length. Calculating expression levels Expression level of ADAR1 and ADAR2 at the human U87MG cell line (with or without siRNA against ADAR1) [14] was calculated using RSEM [64] as either FPKM or transcripts per million. Both measures gave the same fold change between the control and the siRNA samples for both ADAR1 and ADAR2. Direct sequencing validation of hyper-editing To experimentally confirm our computational editing prediction, we chose seven hyper-edited regions and PCR-amplified genomic DNA and cDNA from a human brain from same donor (obtained from the NICHD Brain and Tissue Bank for Developmental Disorders at the University of Maryland, Baltimore, MD, USA). Primers were designed using Primer3 (ref. 65 ). The PCR reaction was performed in C1000 Thermal Cycler (Bio-Rad) using Phusion Green Hot Start II High-Fidelity DNA Polymerase (Thermo Scientific) and in a 20-μl reaction volume, according to the manufacturer’s instructions. We ran the following steps: 98 °C × 30 s, 35 cycles of (98 °C × 10 s, annealing T m°C × 30 s (listed in Supplementary Table 5 ), and 72 °C × 30 s), and 7 min in 72 °C. PCR products were run on a 1% agarose gel, extracted using MinElute gel extraction kit (Qiagen), and sequenced in Hy Laboratories. Chromatograms of matched DNA and cDNA were aligned and editing sites were identified. Counts of observed editing sites in each region appear in Supplementary Table 5 . Annotated chromatograms for two of the regions appear in Supplementary Fig. 3 . How to cite this article: Porath, H. T. et al . A genome-wide map of hyper-edited RNA reveals numerous new sites. Nat. Commun. 5:4726 doi: 10.1038/ncomms5726 (2014).